Intensification of the meridional temperature gradient in the Great Barrier Reef following the Last Glacial Maximum Tropical south-western Pacific temperatures are of vital importance to the Great Barrier Reef (GBR), but the role of sea surface temperatures (SSTs) in the growth of the GBR since the Last Glacial Maximum remains largely unknown. Here we present records of Sr/Ca and δ 18 O for Last Glacial Maximum and deglacial corals that show a considerably steeper meridional SST gradient than the present day in the central GBR. We find a 1–2 °C larger temperature decrease between 17° and 20°S about 20,000 to 13,000 years ago. The result is best explained by the northward expansion of cooler subtropical waters due to a weakening of the South Pacific gyre and East Australian Current. Our findings indicate that the GBR experienced substantial meridional temperature change during the last deglaciation, and serve to explain anomalous deglacial drying of northeastern Australia. Overall, the GBR developed through significant SST change and may be more resilient than previously thought. Sea surface temperature (SST) gradients in the south-western tropical Pacific control the extent of the Western Pacific Warm Pool (WPWP, SST >28 °C), the position and intensity of the Australian summer monsoon and, consequently, hydrological changes on the adjacent continent [1] , [2] . This region hosts the world’s largest extant coral reef, the Great Barrier Reef (GBR) World Heritage Area, with its unique ecosystem that has evolved over hundreds of thousands of years, apparently in response to major environmental perturbations [3] . The SST rise from the Last Glacial Maximum (LGM) to the present is well constrained in the equatorial Pacific Ocean [4] , [5] , [6] , [7] , but is relatively unknown for the unique GBR region. A previous study suggested regional SST changes of ~1.5 °C or less during the late Pleistocene [8] , questioning warming SST as an explanation for the rise of the GBR [9] . However, this result is inconsistent with SST reconstructions for the southeastern Coral Sea [10] and the WPWP [7] that indicate a ~3 °C cooling during the LGM. Clearly, a better understanding of the temperature history of the GBR ecosystem since the LGM is essential in order to establish a baseline against which to judge the potential response of this region to future climate change. Here we investigate the Sr/Ca and δ 18 O environmental proxies in precisely U-Th dated fossil shallow-water corals drilled by Integrated Ocean Drilling Program (IODP) Expedition 325 along the shelf edge seaward of the modern GBR [11] to reconstruct the meridional temperature gradient since the LGM ( Fig. 1 ). Sr/Ca variations in aragonitic coral skeletons are a proxy for SST variability [12] , [13] . However, significant differences in mean Sr/Ca values among corals living on the same reef, and glacial-interglacial changes in seawater Sr/Ca, have hampered the reconstruction of mean tropical SSTs over the last deglaciation [14] , [15] , [16] , [17] , [18] . We circumvent these issues by comparing geochemical averages obtained for a large number of fossil corals from two sites in the GBR. Our premise is that corals from both sites are affected similarly by between-colony offsets, and changes in seawater Sr/Ca, thus allowing us to reconstruct relative changes in the meridional temperature gradient along the GBR. Coral δ 18 O, a proxy that reflects both temperature and seawater δ 18 O variations, and which is affected differently by between-colony offsets in mean coral δ 18 O (refs 19 , 20 ) and glacial-interglacial changes in seawater δ 18 O, is used to support our reconstruction [14] , [21] , [22] . Contrary to coral Sr/Ca, coral δ 18 O can be influenced by site-specific changes in seawater δ 18 O. We show that the meridional SST gradient in the GBR region was considerably steeper than today during the LGM and last deglaciation, which is best explained by northward expansion of cooler subtropical waters, owing to weakening of the South Pacific subtropical gyre and East Australian Current (EAC). Our findings indicate that the GBR experienced substantial and regionally differing temperature change during the last deglaciation, much larger temperature changes than previously recognized. Furthermore, our findings suggest a northward contraction of the WPWP during the LGM and last deglaciation, and serve to explain anomalous drying of northeastern Australia at that time. 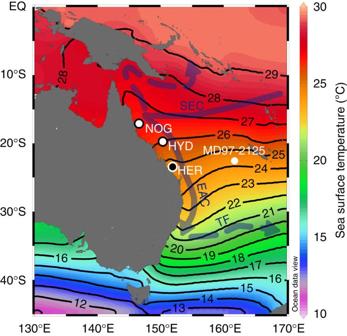Figure 1: Map of the south-western Pacific Ocean. Locations of Integrated Ocean Drilling Program (IODP) Expedition 325 drilling sites at Noggin Pass (NOG) and Hydrographer’s Passage (HYD) in the central Great Barrier Reef11are superimposed on annual mean sea surface temperature35(SST) and surface ocean circulation patterns in the study area39(SEC, South Equatorial Current; EAC, East Australian Current; TF, Tasman Front). For reference, the modern coral site at Heron Island (HER) in the southern Great Barrier Reef and sediment core MD97-2125 in the southeastern Coral Sea10are shown. The Coral Sea is the region off the northeast coast of Australia that is bounded by New Guinea to the north and several smaller islands in the east. The Western Pacific Warm Pool is defined as the region where annual mean SST is greater than 28 °C (ref.62). Figure 1: Map of the south-western Pacific Ocean. Locations of Integrated Ocean Drilling Program (IODP) Expedition 325 drilling sites at Noggin Pass (NOG) and Hydrographer’s Passage (HYD) in the central Great Barrier Reef [11] are superimposed on annual mean sea surface temperature [35] (SST) and surface ocean circulation patterns in the study area [39] (SEC, South Equatorial Current; EAC, East Australian Current; TF, Tasman Front). For reference, the modern coral site at Heron Island (HER) in the southern Great Barrier Reef and sediment core MD97-2125 in the southeastern Coral Sea [10] are shown. The Coral Sea is the region off the northeast coast of Australia that is bounded by New Guinea to the north and several smaller islands in the east. The Western Pacific Warm Pool is defined as the region where annual mean SST is greater than 28 °C (ref. 62 ). Full size image Coral preservation and ages The drill cores of IODP Expedition 325 intersected massive and robust branching/columnar Isopora palifera / cuneata colonies, which are common in shallow-water (0–10 m), high-energy reef crest environments [23] , [24] . Fossil Isopora corals were recovered at Noggin Pass (NOG, 17.1°S) and Hydrographer’s Passage (HYD, 19.7°S) in the central GBR [11] ( Fig. 1 ). The corals were screened for possible diagenetic alteration of their skeletons using X-radiography, powder X-ray diffraction, thin-section petrography and Mg/Ca screening, and are well preserved (Methods and Supplementary Figs 1–4 ). U-Th dating yielded coral ages spanning 25 to 12 thousand years before the present (kyr BP; ‘present’ is defined as AD 1950) (Methods and Supplementary Table 1 ). 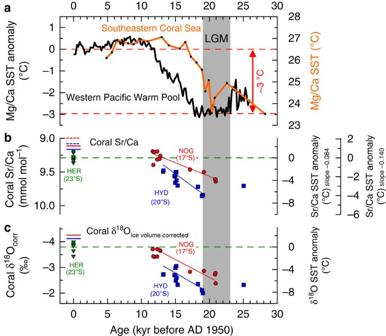Figure 2: Great Barrier Reef coral Sr/Ca and δ18O and western tropical Pacific temperatures. (a) Western Pacific Warm Pool (WPWP) sea surface temperature (SST) anomaly7(leftyaxis) and southeastern Coral Sea SST10(rightyaxis) reconstructed from planktonic foraminiferal Mg/Ca. Modern annual mean WPWP SST is >4 °C warmer than SST in the southeastern Coral Sea35. (b) Mean Sr/Ca of individualIsopora palifera/cuneatacorals from Noggin Pass (NOG) and Hydrographer’s Passage (HYD), central Great Barrier Reef (GBR), and Heron Island (HER), southern GBR (approximate latitude indicated). Weighted least-squares regression lines are shown for NOG and HYD, utilizing data variances as weights. HYD coral Sr/Ca is significantly different from NOG coral Sr/Ca (Methods andSupplementary Fig. 5). The coral-based SST anomalies are not adjusted for changes in seawater Sr/Ca, and thus provide upper estimates of the magnitude of cooling. However, the effects of seawater Sr/Ca changes are similar at both sites, so the reconstructed SST differences between sites are not affected. For reference, the fossil coral-based Sr/Ca-SST anomalies are plotted relative to average Sr/Ca at HER (dashed green line). Modern mean SST35at NOG (26.6 °C) and HYD (26.0 °C) is shown relative to SST at HER (24.5 °C) and scaled using the mean coral Sr/Ca-SST relationships of −0.084 mmol mol−1per °C (ref.34) (solid red and blue lines) and −0.140 mmol mol−1per°C (ref.32) (dashed red and blue lines). (c) As inb, but for mean coral δ18O corrected for the influence of changes in ice volume using a global compilation of benthic foraminifer δ18O records37(for uncorrected coral δ18O seeSupplementary Fig. 8). The resulting coral δ18O-SST anomalies are shown relative to average δ18O at HER (dashed green line) using the average of three mean coral δ18O-SST relationships (−0.22‰ per °C, refs32,33,34). The larger cooling inferred from coral δ18O compared with Sr/Ca suggests a positive seawater δ18O anomaly. Modern mean SST35at NOG and HYD is shown relative to HER (solid red and blue lines). The grey shading indicates the timing of the Last Glacial Maximum63,64(LGM). All coral specimens were analysed for Sr/Ca, δ 18 O, Mg/Ca and δ 13 C along their major growth orientation (Methods; Supplementary Figs 1, 3 and 4 ; Supplementary Table 2 ). A total of 881 samples were analysed at subseasonal resolution in 7 fossil Isopora corals ( Supplementary Fig. 3 ). An additional 18 fossil and 13 modern Isopora were analysed for bulk geochemical composition, as the major aim of the study is the reconstruction of mean SST changes from geochemical averages of corals. Coral-based SST reconstruction The performance of Sr/Ca and δ 18 O in Isopora corals was assessed using modern colonies from Heron Island (HER, 23.4°S) in the southern GBR ( Fig. 1 ), which provides a modern analogue with relatively cool SSTs such as those experienced by last deglacial central GBR corals. The modern corals reveal between-colony offsets in mean Sr/Ca and δ 18 O that are equivalent to ~1–2 °C ( Fig. 2 ) and similar to those seen in Porites corals [18] , [25] ( Supplementary Note 1 ). We note that the modern Isopora corals represent a range of shallow-water habitats on the reef, comparable to the environment represented by the fossil corals. Thus, the between-colony offsets reflect the combined effects of differences in water depth, location on the reef and different time intervals [26] , [27] , [28] . Furthermore, initial comparison of bulk samples from modern Isopora corals from Papua New Guinea, and the central and southern GBR (spanning a mean SST range of ~4.5 °C), indicates similar Sr/Ca-SST and δ 18 O-SST relationships to those for Porites , supporting our use of the better-constrained mean relationships established for Porites (Methods and Supplementary Note 2 ). Figure 2: Great Barrier Reef coral Sr/Ca and δ 18 O and western tropical Pacific temperatures. ( a ) Western Pacific Warm Pool (WPWP) sea surface temperature (SST) anomaly [7] (left y axis) and southeastern Coral Sea SST [10] (right y axis) reconstructed from planktonic foraminiferal Mg/Ca. Modern annual mean WPWP SST is >4 °C warmer than SST in the southeastern Coral Sea [35] . ( b ) Mean Sr/Ca of individual Isopora palifera / cuneata corals from Noggin Pass (NOG) and Hydrographer’s Passage (HYD), central Great Barrier Reef (GBR), and Heron Island (HER), southern GBR (approximate latitude indicated). Weighted least-squares regression lines are shown for NOG and HYD, utilizing data variances as weights. HYD coral Sr/Ca is significantly different from NOG coral Sr/Ca (Methods and Supplementary Fig. 5 ). The coral-based SST anomalies are not adjusted for changes in seawater Sr/Ca, and thus provide upper estimates of the magnitude of cooling. However, the effects of seawater Sr/Ca changes are similar at both sites, so the reconstructed SST differences between sites are not affected. For reference, the fossil coral-based Sr/Ca-SST anomalies are plotted relative to average Sr/Ca at HER (dashed green line). Modern mean SST [35] at NOG (26.6 °C) and HYD (26.0 °C) is shown relative to SST at HER (24.5 °C) and scaled using the mean coral Sr/Ca-SST relationships of −0.084 mmol mol −1 per °C (ref. 34 ) (solid red and blue lines) and −0.140 mmol mol −1 per ° C (ref. 32 ) (dashed red and blue lines). ( c ) As in b , but for mean coral δ 18 O corrected for the influence of changes in ice volume using a global compilation of benthic foraminifer δ 18 O records [37] (for uncorrected coral δ 18 O see Supplementary Fig. 8 ). The resulting coral δ 18 O-SST anomalies are shown relative to average δ 18 O at HER (dashed green line) using the average of three mean coral δ 18 O-SST relationships (−0.22‰ per °C, refs 32 , 33 , 34 ). The larger cooling inferred from coral δ 18 O compared with Sr/Ca suggests a positive seawater δ 18 O anomaly. Modern mean SST [35] at NOG and HYD is shown relative to HER (solid red and blue lines). The grey shading indicates the timing of the Last Glacial Maximum [63] , [64] (LGM). Full size image The fossil coral Sr/Ca-SSTs show the deglacial warming trend for the interval ~21 to ~12 kyr BP ( Fig. 2 ). Furthermore, they show that the deglacial SST rise began no later than 19 kyr BP, consistent with the ~20 kyr BP onset of the deglacial SST rise in the southeastern Coral Sea (MD97-2125; 161°44′E, 22°34′S) [10] ( Figs 1 and 2 ). Importantly, SSTs in the GBR region do not show cooling associated with the Northern Hemisphere Younger Dryas (YD) event [29] (~12.9 to ~11.7 kyr BP). This finding is in contrast to coral Sr/Ca evidence for YD cooling at Vanuatu [16] and Tahiti [17] , located further east, and at the same latitude as the GBR, in the western and central South Pacific. This highlights the regional complexity of the response of low-latitude climates to YD cooling in the North Atlantic region. The relatively warm SSTs in the GBR during the YD are consistent with an Antarctic-type pattern of deglacial warming as observed further to the south [30] , [31] , as well as with the near-continuous deglacial warming observed throughout most of the WPWP to the north [7] . Direct application of modern coral Sr/Ca-SST relationships [32] , [33] , [34] (Methods) would yield estimates of LGM (~21 kyr BP) SSTs 4–6 °C cooler than today at NOG (17°S), and late LGM (~19 kyr BP) SSTs 6–8 °C cooler than today at HYD (20°S). These estimates use modern Isopora corals from HER (23°S) as the modern benchmark and take into account the modern SST difference between HER and the central GBR ( Figs 1 and 2 ). The modern annual mean SSTs are 24.5 °C at HER, and 26.0 °C (HYD) and 26.6 °C (NOG) at the central GBR sites (ref. 35 ). However, the estimates of LGM SSTs are uncorrected for changes in seawater Sr/Ca (owing to large uncertainties in this factor [15] , [17] , [18] ) and are therefore likely to provide upper estimates of the magnitude of cooling. To further constrain the absolute magnitude of SST change, we consider 21.5 °C as the lower limit for coral growth, this temperature being the annual mean SST experienced by modern Isopora corals at Lord Howe Island (159.1°E, 31.5°S), the southernmost Pacific reef [35] , [36] . This ecological constraint implies potential maximum cooling of ~5 °C at NOG and ~4.5 °C at HYD, which is slightly less than the uncorrected coral Sr/Ca-SST estimates, and broadly in line with our understanding of glacial-interglacial changes in seawater Sr/Ca (ref. 15 ). Interestingly, if coral δ 18 O is used on its own to estimate glacial SSTs (correcting for glacial-interglacial changes in seawater δ 18 O (ref. 37 ) but not for regional seawater δ 18 O changes), we find LGM SSTs ~7 °C cooler than today at NOG (17°S) and ~9 °C cooler during the late LGM (~19 kyr BP) at HYD (20°S). Taken together, the apparent 2–4 °C difference between the coral Sr/Ca- and ecologically-based estimate (4–5 °C) and δ 18 O-based estimate (7–9 °C) of LGM SST cooling suggests a positive δ 18 O anomaly (0.4–0.8‰) for GBR surface waters. This anomaly would be consistent with reduced regional precipitation minus evaporation balance at the time, although other changes in the hydrological cycle and surface ocean circulation may also contribute. Coral-based SST gradient reconstruction Our most striking finding is that the mean Sr/Ca values for the 24 fossil Isopora corals with ages spanning ~20 to ~13 kyr BP for the southern (HYD) and northern sites (NOG) form two separate groups ( Fig. 2 ; Supplementary Table 2 ). Regression analysis indicates that the HYD coral Sr/Ca is significantly higher than the NOG coral Sr/Ca (Methods and Supplementary Fig. 5 ). In addition, the significance of the difference between the HYD and NOG palaeo-SSTs is verified by regression analysis of the coral δ 18 O values for the two sites ( Fig. 2 ). Importantly, our analysis of relative changes in the meridional SST gradient is not biased by glacial-interglacial changes in seawater Sr/Ca and δ 18 O because the effects would be essentially the same at both sites. The difference in mean SST changes given by the HYD and NOG coral Sr/Ca and δ 18 O indicates that the southern site was on average 2–3 °C cooler [32] , [33] , [34] relative to the northern site from ~20 to ~13 kyr BP ( Fig. 2 ). Given the relatively small meridional difference in SST today (<0.6 °C, ref. 35 ; Supplementary Discussion) between the two sites ( Fig. 1 ), our results indicate a steeper meridional SST gradient along the central GBR between 17° and 20°S throughout most of the LGM and deglaciation. Today, meridional SST gradients such as those along the GBR during the LGM and deglaciation are only observed south of ~30°S on the eastern Australian margin [35] ( Fig. 1 ). At this latitude, the EAC, which transports warm tropical waters southward along the eastern Australian coast, separates from the continent to form the Tasman Front [38] , [39] . Therefore, the steeper LGM and deglacial SST gradient may be due to EAC weakening and northward expansion of cooler subtropical waters. Furthermore, the relatively high δ 18 O of central GBR waters during the LGM, shown by the coral records, supports the interpretation of northward expansion of high-salinity subtropical waters ( Supplementary Fig. 6 ). The results are consistent with studies of planktonic foraminifer assemblages [40] and δ 18 O (ref. 38 ), indicating northward displacement of subtropical waters, the EAC separation and the Tasman Front to ~25°S during the LGM [40] and deglaciation [38] . However, our results indicate that cooler waters were displaced as far north as 20° to 17°S in the central GBR, and that the steeper meridional SST gradient at this latitude was a robust feature of the LGM and deglaciation. The coral Sr/Ca data indicate that the SST gradient decreased significantly from the LGM towards the late deglaciation ( Fig. 2 ; Supplementary Fig. 5 ), due to greater warming at the southern site compared with the northern site. The available palaeoclimate records indicate that the steeper meridional SST gradient in the central GBR does not reflect a regionally steeper meridional SST gradient in the south-western tropical Pacific because the south-western tropical Pacific meridional SST gradient was actually weaker than today during the last deglaciation. The deglacial SST rise in the southeastern Coral Sea (MD97-2125; 161°44′E, 22°34′S) started earlier (~20 kyr BP) and reached modern SST as early as ~17 kyr BP (ref. 10 ), whereas warming in the WPWP commenced at ~17.5 kyr BP and reached modern SST as late as ~12 kyr BP (ref. 7 ) ( Fig. 2 ). Both regions cooled by similar amounts during the LGM (~3 °C) (refs 7 , 10 ) and today the WPWP is >4 °C warmer than the southeastern Coral Sea [35] ( Figs 1 and 2 ), so the earlier start of the deglacial warming in the southeastern Coral Sea, relative to warming in the WPWP, means that the meridional SST gradient in the tropical southwest Pacific was weaker than today during the last deglaciation. This is opposite to our reconstructed steepening of the meridional SST gradient along the central GBR at that time, and is consistent with weakening of the EAC along the eastern Australian coast during the LGM and deglaciation. Furthermore, the reduction in heat transfer from low to mid-latitudes due to weakening of the EAC, which is the western boundary current of the South Pacific subtropical gyre, may have played an important role in dampening the amplitude of LGM cooling in the WPWP. Interestingly, the increase in heat transfer from low to mid-latitudes implied by EAC strengthening after ~12.7 kyr BP, suggested by the coral records, coincides with the end of the deglacial SST rise in the WPWP [7] . The results suggest an important role for variations in the strength of the South Pacific’s western boundary current, and changes in the transport of warm tropical waters to higher latitudes, in contributing to SST changes in the WPWP on glacial-interglacial timescales. A steeper meridional SST gradient and cooler ocean surface off northeast Australia between ~20 and ~13 kyr BP may explain anomalously dry conditions in northeastern Australia at that time inferred from the Lynch’s Crater sediment record [1] , [41] (145°70′E, 17°37′S). The cooler deglacial waters could have reduced the effectiveness of the southeasterlies in advecting moisture from the Coral Sea to the adjacent continent. Furthermore, these waters could have potentially restricted the southern boundary of the WPWP and southward migration of the Intertropical Convergence Zone to a more northerly position, thus inhibiting development of the Australian summer monsoon. The southward displacement of subtropical waters after ~12.7 kyr BP, indicated by the coral records, was potentially accompanied by a southward shift of the southern boundary of the WPWP and the Intertropical Convergence Zone, and was probably driven by spin-up of the South Pacific subtropical gyre and corresponding strengthening of the EAC in response to deglacial warming [38] . Our findings indicate that the GBR has experienced much larger SST changes—both spatially and temporally—since the LGM than previously recognized. This was especially the case in the south, owing to significant steepening of the meridional SST gradient resulting from a northward expansion of cooler subtropical waters during the LGM and deglaciation. Combined with evidence for the existence of extensive reefs along the shelf edge seaward of the modern GBR at that time [11] , [42] , our results provide new insights into the ability of coral reefs to adapt to temperature change. Most corals are well adapted to their local temperature regime, but are susceptible to thermal stress resulting in bleaching and sometimes mortality, where the mean summer maximum temperature is exceeded by >~1 °C (ref. 43 ). As a consequence, the absolute thermal limit for coral bleaching is strongly site dependent [43] , and questions remain on the timescales over which corals may adapt to temperature rise [44] , [45] . The apparent resilience of the GBR Isopora coral reef community throughout much of the last deglaciation, despite substantial increases in SST from the LGM condition, demonstrates that adaption occurred over a few thousand years or less. This apparent resilience further suggests that, considering temperature alone, southward expansion of this robust reef crest community could be an important response to future climate warming. Coral samples Fossil Isopora palifera / cuneata corals were recovered in 2010 by IODP Expedition 325 off the central Great Barrier Reef [11] (GBR). Corals were recovered at depths between 56 and 126 m below modern sea level at Noggin Pass (NOG; 146.6°E, 17.1°S; IODP sites M0053 and M0057) and Hydrographer’s Passage (HYD; 150.3°E, 19.7°S; IODP sites M0031, M0033, M0035, M0036 and M0039) using the mission-specific platform ‘Greatship Maya’. Modern Isopora palifera / cuneata corals were collected at Heron Island (HER; 151.9°E, 23.4°S) in the southern GBR from 1974 to 1979 at depths between 0 and 14 m. Screening for diagenesis The aragonitic skeletons of all fossil corals were analysed by powder X-ray diffraction and X-radiography, indicating ≤1.5% calcite ( Supplementary Table 2 ) and demonstrating that skeletal areas of obvious diagenetic alteration were not analysed ( Supplementary Fig. 1 ). Selected fossil corals were also investigated using petrographic thin sections and showed excellent preservation of primary porosity, with no evidence for significant amounts of secondary aragonite or calcite cements ( Supplementary Fig. 2 ). Skeletal Mg/Ca ratios indicate the absence of significant amounts of high-Mg calcite and secondary aragonite cements along the analysed transects ( Supplementary Figs 3 and 4 ). Seven corals were analysed at 0.3-mm resolution for element/Ca and stable isotope ratios. No influence of subtle diagenetic alteration was detected on this spatial scale. The reported mean geochemical values are very similar to those for corals of similar age analysed for bulk composition. U-Th dating The chronology of the fossil corals was determined by U-Th dating carried out using different methods at three laboratories: Woods Hole Oceanographic Institution (WHOI), Australian National University (ANU) and University of Oxford (OX). The originating laboratories are identified alongside the data in Supplementary Table 1 . U-Th ages are reported in kyr before the present relative to AD 1950. Interlaboratory replicate age determinations for a single specimen agree to within 100 years, which is similar to the intra-coral variability observed in some specimens measured using the high-precision (WHOI) method. The corals used in this study have initial 234 U/ 238 U activity ratios between 1.140 and 1.150, which are close to the modern seawater composition giving additional confidence in the chronology. Briefly the methods are: At WHOI, U and Th isotopes are measured by MC-ICP-MS in static mode with all isotopes in Faraday collectors [46] . Large ~5-g subsamples of coral are dissolved and spiked with a mixed 233 U: 236 U: 229 Th tracer, optimized for deglacial age samples and co-precipitated with Fe. To determine the 230 Th/ 238 U, purified U and Th fractions are recombined such that U and Th are measured together at isotope ratios that can be closely matched to bracketing standards. The 234 U/ 238 U is similarly determined statically in Faraday collectors but on an unspiked aliquot. At ANU, U and Th isotopes are measured by thermal ionization mass spectrometry (ref. 47 ). Approximately 1–2 g of coral samples are spiked with a mixed 233 U: 229 Th tracer, and U and Th are separated using U-Teva resin in a single pass. The 229-230-232 Th isotopes were measured simultaneously in charge mode, in Faraday cups, using 20 pF feed-back capacitors as active electrometer elements [48] . U isotopes 233-234-235 U are also measured in charge-collection mode while, 238 U is measured using a 10 10 -Ohm feed-back resistor simultaneously in Faraday cups. The magnitude of the 238 U low-mass tail was monitored continuously at mass 237 U in charge mode. This was used to subtract the 238 U tail from under 233-234-235 U isotopes. Extensive measurements with an unspiked U-standard HU-1 showed that the curvature of the 238 U tail remained invariant under a wide range of operating conditions, in particular, at the expected locations of the 233-236 U peaks. U sample loads, on single rhenium filaments, ranged from 0.5 to 0.8 μg and the 238 U beam intensity was kept between 8 × 10 11 and 10 × 10 11 A for several hours. At these intensities, the 10 10 -Ohm feed-back resistor was used to avoid response-time problems encountered with the considerably slower 10 11 -Ohm resistors. The instrument was calibrated with reference to a secular equilibrium standard HU-1. Comparisons with Western Australian coral samples for the last interglacial [47] showed precise agreement with previous measurements. At OX, U and Th isotopes are measured by MC-ICP-MS utilizing ion counter collectors for the minor isotope beams. Approximately 0.3 g of coral samples are dissolved and spiked with a mixed 236 U: 229 Th tracer. U and Th are purified and measured separately: U isotopes, statically; and Th by peak hopping the 229 and 230 beams into an ion counter normalizing beam intensity between steps with either 232 Th or 235 U measured in Faraday collectors. Instrumental biases and relative collector efficiencies are accounted for using standard-sample bracketing using U and Th isotope standards [49] . All activity ratios and ages are calculated using the half lives reported in ref. 50 . Ages are presented in Supplementary Table 1 as ‘raw’, assuming all 230 Th is accumulated in the coral since growth, and an age corrected for detrital 230 Th. The detrital correction makes use of the measured 232 Th/ 238 U as a proxy for the amount of detrital contamination, an assumed detrital composition of crustal origin [51] , and an allowance for non-secular equilibrium of the contaminant ( 232 Th/ 238 U=1.21±0.6, 230 Th/ 238 U=1±0.25 and 234 U/ 238 U=1±0.25). All ages are calculated relative to AD 1950 for consistency. Microsampling All coral specimens were microsampled continuously along their major growth orientation ( Supplementary Fig. 1 ). We note that the major growth axis of a coral colony is difficult to discern from drill cores with a diameter much smaller than the colony, and that sampling paths with respect to coral morphology may produce different geochemical variations [52] , [53] , [54] . We cannot completely exclude such effects but note that the majority of our massive Isopora specimens indicate uniform parallel growth of corallites, suggesting the absence of colony morphology effects on this spatial scale. Seven corals were microsampled at subseasonal resolution, by milling a trench 2.4 mm wide and 3.0 mm deep, using a sample-step increment of 0.3 mm. All other corals were sampled for bulk geochemical composition by milling a continuous trench of similar width and depth. Geochemical and isotopic analyses Coral element/Ca and stable isotope ratios were analysed on splits of the same sample powders at MARUM (Bremen), ANU (Canberra), LDEO (Palisades), GeoSciences (Edinburgh), AIST (Tsukuba) and AORI (Kashiwa), using ICP-OES, ICP-MS and dual-inlet stable-isotope ratio mass spectrometry. Bulk powders of fossil corals were analysed at least in triplicate. The coral reference material JCp-1 was used to correct for interlaboratory offsets [55] . The JCp-1 reference compositions used in this study are 8.781 mmol mol −1 for Sr/Ca, −4.75‰ for δ 18 O, 4.252 mmol mol −1 for Mg/Ca and −1.58‰ for δ 13 C. These values represent the average of >100 element/Ca and >60 δ 18 O and δ 13 C analyses of splits of JCp-1 powder that were treated like samples in the participating laboratories. Isopora coral as an SST archive Isopora [56] has been considered a subgenus of the coral genus Acropora , but was recently elevated to genus [57] . Massive and robust branching/columnar Isopora palifera/cuneata corals are common in the upper 10 m of well-flushed reef crest environments [23] , [24] , providing an excellent potential archive of open-ocean SST. However, submillimetre-scale analysis of seven massive Isopora , the growth form most common in our study, did not reveal clear annual cycles in Sr/Ca and δ 18 O ( Supplementary Fig. 3 ). It is possible that the complex skeletal architecture, including discontinuous filament-like structures perpendicular to the growth direction, and spatially heterogeneous calcification processes within massive Isopora corals obscure the annual cycle given that diagenesis was ruled out for these samples. We note that studies on branching Acropora corals ( A. palmata , A. nobilis ) did not reveal clear annual cycles in Sr/Ca and δ 18 O along axes of radial growth [58] , [59] , which was attributed to spatially heterogeneous calcification processes such as secondary thickening of skeletal elements [58] , [59] , [60] . In the absence of definitive calibration data for massive Isopora , the average of well-established mean proxy-SST relationships for Porites corals was used to reconstruct changes in mean SST: −0.084 mmol mol −1 per °C (ref. 34 ), −0.089 mmol mol −1 per °C (ref. 33 ), −0.140 mmol mol −1 per °C (ref. 32 ) for coral Sr/Ca and −0.22‰ per °C (refs 32 , 33 , 34 ) for coral δ 18 O. The relationships for Porites are based on rescaled seasonal calibrations for studying changes in mean SST [34] , on calibrations derived from bulk coral values for reef settings with different average temperatures [33] and on annual mean calibrations using coral time series [32] . Preliminary bulk calibration experiments on modern Isopora corals suggest similar Sr/Ca- and δ 18 O-SST relationships to the better-studied Porites genera ( Supplementary Fig. 7 ; Supplementary Note 2 ). The Isopora bulk calibration slope for Sr/Ca lies closer to the seasonal Porites slope for Sr/Ca than to the bulk Porites slope. Furthermore, seasonal Sr/Ca calibration slopes similar to Porites were reported for a coral in the same family as Isopora , Acropora palmata [58] , and early studies found similar Sr/Ca and δ 18 O bulk calibration slopes for Acropora and Porites [26] , [27] . For the fossil Isopora corals, the subseasonally resolved geochemical records and analysis of density bands in X-radiographs (subseasonally and bulk-sampled corals) indicate that each coral analysed encompasses several years of skeletal growth. On the basis of this anaylsis, there is no clear indication for systematically lower growth rates at the southern site compared with the northern site. Thus the relatively cool reconstructed SSTs at the southern site are not the result of a potential influence of lower growth rates on SST proxies. Statistical analysis Regression analysis was performed by applying a straight-line weighted least-squares fit (utilizing data variances as weights, 1/sigma(i) [2] , ref. 61 ) to the coral data from HYD and NOG and the difference in straight-line fit (HYD−NOG) was determined. A Monte Carlo error simulation [61] was performed for the difference in straight-line fit by generating random deviations from original data points, from which simulated straight lines and simulated fit differences resulted. The s.e. of these differences (versus time) was used to generate the error envelope ( Supplementary Fig. 5 ). Simulations (400) were performed with independent, normally distributed random deviations (s.d. equal to dating error for age simulation and equal to measurement error × inflation factor for proxy simulation). The fit residuals were used to determine the mean deviation from the fitted line (root of residual mean square). This quantity was compared with the mean proxy measurement error, which is smaller by a factor of 2 for HYD coral δ 18 O, smaller by a factor of 3 for NOG coral δ 18 O, smaller by a factor of 2 for HYD coral Sr/Ca and about the same for NOG coral Sr/Ca. Consequently, a conservative approach was chosen by artificially inflating the assumed measurement error, in order to simulate the influence of errors induced by effects such as between-colony variability. A measurement-error inflation factor of 3.0 was used to calculate the s.e. band for our difference in straight-line fit. However, the difference is still larger than zero for both coral Sr/Ca and δ 18 O. Therefore the HYD coral Sr/Ca is significantly different from the NOG coral Sr/Ca, and the HYD coral δ 18 O is significantly different from the NOG coral δ 18 O. How to cite this article: Felis, T. et al . Intensification of the meridional temperature gradient in the Great Barrier Reef following the Last Glacial Maximum. Nat. Commun. 5:4102 doi: 10.1038/ncomms5102 (2014).